Retrieving the intracellular topology from multi-scale protein mobility mapping in living cells In living cells, most proteins diffuse over distances of micrometres within seconds. Protein translocation is constrained due to the cellular organization into subcompartments that impose diffusion barriers and guide enzymatic activities to their targets. Here, we introduce an approach to retrieve structural features from the scale-dependent mobility of green fluorescent protein monomer and multimers in human cells. We measure protein transport simultaneously between hundreds of positions by multi-scale fluorescence cross-correlation spectroscopy using a line-illuminating confocal microscope. From these data we derive a quantitative model of the intracellular architecture that resembles a random obstacle network for diffusing proteins. This topology partitions the cellular content and increases the dwell time of proteins in their local environment. The accessibility of obstacle surfaces depends on protein size. Our method links multi-scale mobility measurements with a quantitative description of intracellular structure that can be applied to evaluate how drug-induced perturbations affect protein transport and interactions. Cellular structures such as membranes, chromatin, cytoskeleton and cytoplasmic organelles form a dynamic three-dimensional maze through which proteins have to find their way to reach the sites where they are active. The topology of the cellular interior is a key factor for target search processes and enzymatic reactions [1] that are the basis for cell function. To map the properties of dynamic structures like chromatin in living cells as they are ‘sensed’ by a diffusing protein, direct visualization of all cellular constituents at high spatial and temporal resolution is needed. Currently, cryo-electron microscopy enables three-dimensional imaging of cellular structures at molecular resolution [2] but has the drawback that it is only applicable to fixed samples. Recent advances in super-resolution light microscopy allow for mapping labelled structures in living cells with sub-diffraction resolution of ~20 nm (ref. 3 ). However, they do not provide the temporal resolution required to follow fast molecular translocations. A complementary approach that is well established in the field of diffusion NMR is it to infer structural information from the mobility of an inert nanosensor that explores the accessible space of a structure [4] , [5] , [6] , [7] . This strategy has been successfully applied to investigate pore sizes and connectivity in rocks, clays and biological tissues [4] , [7] , [8] . Here, we introduce this concept to fluorescence correlation spectroscopy (FCS) to link protein mobility and cellular structure in single cells at high resolution [9] , [10] , [11] . To this end, we map the mobility of inert monomers, trimers and pentamers of the green fluorescent protein (GFP) domain on multiple length and time scales in the cytoplasm and nucleus by parallelized FCS measurements with a line-illuminating multi-focus fluorescence microscope. With drugs specifically targeting different cellular components we investigate how perturbations of the cellular structure affect protein transport. Furthermore, we compare the mobility of inert GFP multimers to GFP fusions of the signal transducer and activator of transcription 2 (STAT2) protein and the chromodomain of heterochromatin protein 1 beta (HP1β). From the perspective of these proteins that cover the size range of most enzymes, the cellular interior appears as a porous medium made up by randomly distributed obstacles with characteristic size and density. Its structure reorganizes in response to intra- and extracellular cues and acts as a viscous medium on large molecules, while it partitions the cellular content for smaller molecules. Protein mobility maps mirror the intracellular architecture Cellular structures reduce molecular mobility in a time- and length-scale-dependent manner. Thus, mobility maps acquired on multiple scales contain hidden information on the cellular environment. To be able to simultaneously measure protein translocations with microsecond time resolution on multiple length scales from 0.2 to ~3 μm, we extended the principle of FCS measurements at a single point in the sample to simultaneous FCS measurements at hundreds of positions arranged along a line. For this purpose, we used a line-illuminating confocal microscope with parallel fluorescence signal acquisition from several hundred detection volumes positioned within the cell, where each detection volume corresponds to a pixel of an electron multiplying charge-coupled device (EM-CCD) detector array ( Fig. 1a ). This setup was previously introduced as a spatial and temporal fluctuation microscope (STFM) [12] and was further developed for the applications described here. When operated in the conventional FCS mode, fluorescence intensity fluctuations at each pixel can be evaluated with an auto-correlation (AC) analysis to obtain spatially resolved mobility and concentration profiles. In addition to parallelized AC measurements, the simultaneously recorded fluorescence signals can be used for fluorescence cross-correlation spectroscopy (FCCS) experiments: Cross-correlation (XC) analysis of signals from different detection volumes yields the diffusion coefficients for transport between selected positions along the line in living cells. Since this can be done for all combinations of the detection elements at the same time, thousands of XC functions can be obtained in a single experiment. For each distance between detection volumes, the diffusion coefficient is determined on the corresponding length and time scale. Simultaneous measurement of the diffusion coefficient on multiple scales allows for reconstructing the environment in which the transport process under study takes place ( Fig. 1b ). The approach described here to conduct this type of analysis is referred to as multi-scale FCCS (msFCCS). The resulting set of AC and XC curves obtained by msFCCS can be visualized as correlation carpets ( Fig. 1c ): Each column of the carpet represents a color-coded correlation curve as shown for idealized AC and XC carpets in homogeneous solution. AC carpets are simply the AC functions ‘attached’ vertically to each pixel along the horizontal axis that represents the detection line. XC carpets are obtained by computing XC curves for each pixel correlated with another pixel that is separated along the line by a fixed distance. The resulting XC curves are then assigned to the pixel in the center between the two cross-correlated positions. In this manner, XC carpets can be generated for every possible pixel distance, with the AC carpet being the special case of zero distance. Pixel combinations that include diffusion barriers and lack molecule exchange appear as gaps with low correlation amplitudes. This has been demonstrated earlier via the analysis of spatial pair-correlation functions [13] obtained with scanning FCS setups that have been particularly useful for studying protein lateral diffusion in cell membranes [14] , [15] , [16] . In comparison to scanning-based techniques, the msFCCS approach benefits from complete spatio-temporal coverage. Along the measurement line, there are neither spatial nor temporal gaps for data acquisition and all combinations of lag time and displacement contribute to the calculated high-resolution XC curves. 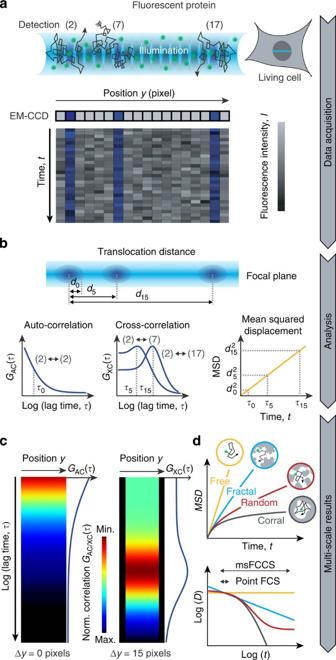Figure 1: Parallelized acquisition of fluorescence signals for msFCCS analysis. (a) Line illumination and parallelized multifocal fluorescence signal detection. Fluorescent proteins enter and leave the detection volumes by diffusion. The resulting local fluctuations in the fluorescence signal are detected on corresponding pixels of an EM-CCD camera array. (b) AC and XC analysis. By applying correlation analysis to the fluorescence signal recorded at a given detector pixel, AC curves can be calculated at every pixel position. Correlation of signals from spatially separated detection volumes are evaluated by computing XC curves (for example, signals of detection volumes 2 and 7 or detection volumes 2 and 17). These yield the MSD, the diffusion coefficientDand the concentration or molecule transmission rate as a function of the translocation distancednor translocation timeτn. (c) AC curves or XC curves for a constant distance between detection elements are acquired along the illumination line and are visualized in so-called correlation carpets, from which diffusion barriers can be identified. (d) The diffusion coefficients determined for different distances can be used to reconstruct the molecules’ MSD as a function of the diffusion timet. The time dependence of the diffusion coefficient reflects the nanostructure ‘seen’ by the diffusing protein. Norm, normalized. Figure 1: Parallelized acquisition of fluorescence signals for msFCCS analysis. ( a ) Line illumination and parallelized multifocal fluorescence signal detection. Fluorescent proteins enter and leave the detection volumes by diffusion. The resulting local fluctuations in the fluorescence signal are detected on corresponding pixels of an EM-CCD camera array. ( b ) AC and XC analysis. By applying correlation analysis to the fluorescence signal recorded at a given detector pixel, AC curves can be calculated at every pixel position. Correlation of signals from spatially separated detection volumes are evaluated by computing XC curves (for example, signals of detection volumes 2 and 7 or detection volumes 2 and 17). These yield the MSD, the diffusion coefficient D and the concentration or molecule transmission rate as a function of the translocation distance d n or translocation time τ n . ( c ) AC curves or XC curves for a constant distance between detection elements are acquired along the illumination line and are visualized in so-called correlation carpets, from which diffusion barriers can be identified. ( d ) The diffusion coefficients determined for different distances can be used to reconstruct the molecules’ MSD as a function of the diffusion time t . The time dependence of the diffusion coefficient reflects the nanostructure ‘seen’ by the diffusing protein. Norm, normalized. Full size image To evaluate how a fluorescent particle ‘senses’ the obstacle density and the organization of the local environment ( Fig. 1d ), the mean squared displacement (MSD) and the corresponding time dependence of the diffusion coefficient were calculated from sets of AC and XC carpets optained by msFCCS. By applying Supplementary Equation (31) for a given pixel pair, an effective diffusion distance is calculated. It corresponds to the mean distance travelled by a molecule when detected in the first and subsequently in the second pixel, and an effective diffusion time calculated according to Supplementary Equation (32) that is approximately represented by the maximum of the XC function ( Fig. 1b ). The effective diffusion distances and times can readily be transformed into the MSD and the time-dependent diffusion coefficient D ( t ) profile. In aqueous solution without obstacles, normal diffusion is observed, for which the diffusion coefficient is time-independent and the MSD scales linearly with time ( Fig. 1d ). In the presence of a significant concentration of obstacles, the mobility is reduced in a scale-dependent manner that is referred to as anomalous diffusion [17] , [18] . This mobility reduction is caused by collisions and binding reactions of particles with their cellular environment, which depend on the specific nature of the tracer molecule. Besides hydrodynamic effects, interactions between particles and obstacles can involve ‘simple’ hard sphere repulsion modulated by electrostatic and van-der-Waals’ interactions as well as more long-lived binding reactions. Thus, D ( t ) represents an apparent diffusion coefficient that includes information on the obstacle network encountered by a diffusing protein. To dissect the structural features of its environment, it is informative to visualize the scale-dependent diffusion coefficient D ( t ) in a double-logarithmic plot versus translocation time t ( Fig. 1d ). For inert tracer molecules and an accessible space with fractal geometry [19] , [20] , the diffusion coefficient follows a straight line in double-logarithmic representation. For random porous geometries, it is a sigmoidal-shaped function [7] , [21] . For very high obstacle densities, the molecules get trapped leading to corralled movements within a confined region [22] . Since our setup uses continuous line illumination, neighbouring pixels have overlap in the fluorescence signal they record. This results in an AC-type pseudo-correlation contribution for XC curves at short distances. To account for this contribution, a detailed characterization of the microscope’s point-spread function (PSF) was carried out ( Fig. 2a ; Supplementary Notes 1 and 2 ; Supplementary Figs 1–3 ; Supplementary Tables 1 and 2 ). Instead of the commonly used three-dimensional Gaussian function, we implemented a double-cone shaped model function [23] for the PSF that provides a more accurate description ( Supplementary Note 1 ). Slow-intensity fluctuations due to large-scale movements of cellular components and out-of-focus fluorescence bleaching were removed by Fourier filtering ( Fig. 2b ; Supplementary Note 3 ; Supplementary Figs 4–6 ). Instrumental setup and data analysis pipeline were validated with reference measurements of inert quantum dots (QDots) and TetraSpeck beads in buffer to ensure that the experimental XC curves were described accurately by the theoretical model functions for all detection volumes and correlation distances ( Fig. 2c–e ; Supplementary Note 4 ). The absolute diffusion coefficients obtained in these experiments were in excellent agreement with literature values ( Table 1 ). 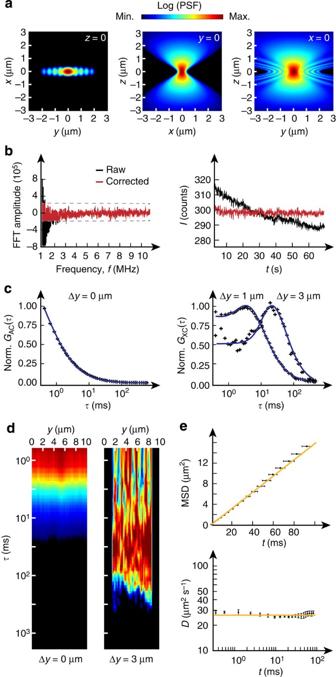Figure 2: Instrument characterization, signal processing and validation of the data analysis pipeline. (a) Approximation of the PSF of the line-confocal microscope as used for subsequent correlation analysis. (b) Fluorescence signal correction by Fourier filtering. Left: exemplary raw and corrected Fourier transformed fluorescence signal in the frequency domain. Right: fluorescence signal before and after signal correction in the time domain. (c) Experimental AC curve and XC curves for 1 and 3 μm diffusion distance for a reference measurement with 20 nM QDots in aqueous solution. Correlation curves were fitted withSupplementary Equation (22). (d) Experimental AC and XC carpet (3 μm) of QDots measured in water. (e) The MSD scales linearly with time for the QDot reference measurements in water as expected for free diffusion. Data are mean values ±s.e.m. (n=10 measurements). Norm., normalized. Figure 2: Instrument characterization, signal processing and validation of the data analysis pipeline. ( a ) Approximation of the PSF of the line-confocal microscope as used for subsequent correlation analysis. ( b ) Fluorescence signal correction by Fourier filtering. Left: exemplary raw and corrected Fourier transformed fluorescence signal in the frequency domain. Right: fluorescence signal before and after signal correction in the time domain. ( c ) Experimental AC curve and XC curves for 1 and 3 μm diffusion distance for a reference measurement with 20 nM QDots in aqueous solution. Correlation curves were fitted with Supplementary Equation (22) . ( d ) Experimental AC and XC carpet (3 μm) of QDots measured in water. ( e ) The MSD scales linearly with time for the QDot reference measurements in water as expected for free diffusion. Data are mean values ±s.e.m. ( n =10 measurements). Norm., normalized. Full size image Table 1 Mobility parameters obtained for different tracer molecules in vitro and in the nucleus of living cells. Full size table Permeability maps show local structural heterogeneity The mobility of inert GFP monomers (GFP 1 ), trimers (GFP 3 ) and pentamers (GFP 5 ) was measured in the nucleus and cytoplasm of human U2OS cells. As a reference, the mobility of GFP 1 was also determined in aqueous solution. The msFCCS curves were acquired at about 50 positions that were equally distributed along a line of 10 μm in length. In aqueous solution, the diffusion coefficients of GFP 1 were independent of the translocation distance, with increasing s.d. due to decreasing signal-to-noise ratios at larger distances ( Fig. 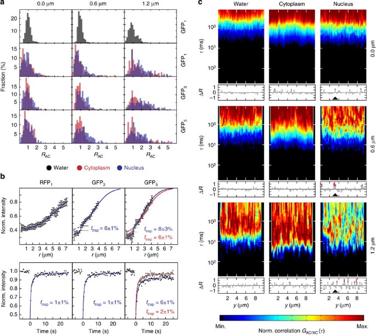Figure 3: Diffusion coefficients, trapped protein fractions and diffusion barrier density determined for GFP in living cells. (a) Histograms for the retardation coefficientRAC=DAC/D(n>200 values). The parameterRACcorresponds to the translocation time of GFP monomer (GFP1), trimer (GFP3) and pentamer (GFP5) molecules relative to the average value obtained from the AC analysis. Measurements were conducted at about 50 positions equally distributed on a 10 μm long line for separation distances of 0 μm (AC), 0.6 μm and 1.2 μm (XC) in water, the nucleus and the cytoplasm. (b) FRAP measurements of RFP1(n=12 cells), GFP3(n=13 cells) and GFP5(n=12 cells). The fraction of trapped proteinftrapwas obtained from the fit of either the post-bleach radial intensity profile after 100 ms withSupplementary Equation (29)(top row) or the average recovery curve withSupplementary Equation (30)(bottom row). Diffusion coefficients were determined from the average recovery curves. Data are mean values, error bars represent s.e.m. (c) Representative AC and XC carpets (0 μm, 0.6 μm and 1.2 μm separation distance) for GFP1in water, nucleus and cytoplasm. Regions with diffusion barriers can be identified from the fold increase of the translocation time ΔRplotted below the carpets. Negative ΔRvalues correspond to a decrease of the translocation time. An example for a diffusion barrier that is most pronounced for the 0.6 μm separation distance is marked with an arrowhead. Norm., normalized. 3a and Supplementary Table 3 ). In contrast, diffusion coefficients of GFP 1 , GFP 3 and GFP 5 in the cytoplasm and nucleus decreased with increasing separation distance. This demonstrates that the diffusion process in cells was significantly slowed down in a length-scale-dependent manner and deviated from free diffusion. The mobility histograms for larger translocation distances were broadened and showed an increasing fraction of proteins with reduced mobility as compared with that measured on short time scales. Thus, the cellular interior appeared heterogeneous and some particles became at least transiently trapped. To quantitate the amount of trapped particles, we conducted complementary fluorescence recovery after photobleaching (FRAP) experiments ( Fig. 3b and Supplementary Note 5 ). 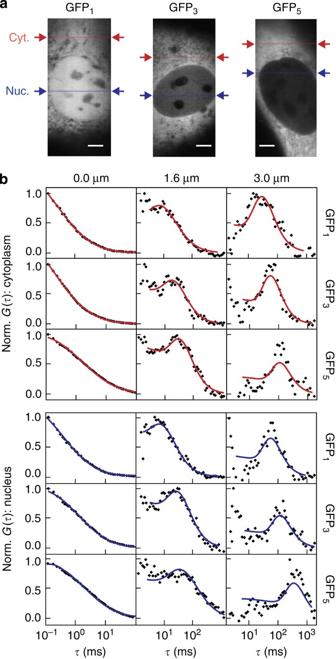Figure 4: Measurements on multiple length scales by msFCCS. (a) Line-confocal fluorescence images of representative U2OS cells expressing GFP1, GFP3and GFP5. The line positions for the measurement of AC and spatial XC functions in homogeneous regions of the nucleus and cytoplasm are indicated. (b) Representative average AC (0 μm) and XC (1.6 and 3 μm) curves obtained in cytoplasm (red) and nucleus (blue). For large diffusion distances, distinct peaks were visible in the diffusion time distributions that shift to larger translocation times for increasing diffusion distance. Solid lines represent the fitted model functions given bySupplementary Equation (22). Scale bar, 5 μm. Cyt, cytoplasm; Nuc, nucleus; Norm, normalized. We first evaluated the post-bleach radial intensity profile [24] that yielded information about particles trapped for at least 100 ms ( Supplementary Table 4 ). As a reference monomeric red fluorescent protein (RFP 1 ) was measured simultaneously with GFP 3 ( r H ≈5.5 nm) and GFP 5 ( r H ≈7.9 nm). RFP 1 has a similar hydrodynamic radius to GFP 1 ( r H ≈2.8 nm) and can be spectrally separated from GFP 3 and GFP 5 . Thus, it is a convenient internal standard to exclude experimental artifacts that might originate from focus drift, optical aberrations or cell motion. The amount of RFP 1 that was trapped for at least 100 ms in the nucleus was negligible ( Fig. 3b ). In contrast, significant fractions of about 6–8% trapped GFP 3 and GFP 5 were present ( Supplementary Table 4 ). To quantitate the amount of molecules trapped for at least 1 min, we conducted a conventional FRAP analysis of the average recovery curve that yielded hardly any trapped GFP 5 in the cytoplasm, while the immobile fraction of GFP 5 in the nucleus persisted. This suggests that the throat size χ of small pores that confine GFP 5 is similar to the hydrodynamic diameter of GFP 5 , which equals 15.8 nm. In the nucleus, these throats seem to remain closed on the minute time scale, whereas corresponding regions in the cytoplasm open up faster so that trapping is detected only on the 100-ms time scale. The diffusion coefficients of RFP 1 , GFP 3 and GFP 5 determined by FRAP using a bleach spot with a radius of 1.3 μm were in good agreement with the values obtained here by msFCCS ( Table 1 ) and the values obtained recently by pixel-wise photobleaching profile evolution analysis [25] on the same length scale. Figure 3: Diffusion coefficients, trapped protein fractions and diffusion barrier density determined for GFP in living cells. ( a ) Histograms for the retardation coefficient R AC = D AC / D ( n >200 values). The parameter R AC corresponds to the translocation time of GFP monomer (GFP 1 ), trimer (GFP 3 ) and pentamer (GFP 5 ) molecules relative to the average value obtained from the AC analysis. Measurements were conducted at about 50 positions equally distributed on a 10 μm long line for separation distances of 0 μm (AC), 0.6 μm and 1.2 μm (XC) in water, the nucleus and the cytoplasm. ( b ) FRAP measurements of RFP 1 ( n =12 cells), GFP 3 ( n =13 cells) and GFP 5 ( n =12 cells). The fraction of trapped protein f trap was obtained from the fit of either the post-bleach radial intensity profile after 100 ms with Supplementary Equation (29) (top row) or the average recovery curve with Supplementary Equation (30) (bottom row). Diffusion coefficients were determined from the average recovery curves. Data are mean values, error bars represent s.e.m. ( c ) Representative AC and XC carpets (0 μm, 0.6 μm and 1.2 μm separation distance) for GFP 1 in water, nucleus and cytoplasm. Regions with diffusion barriers can be identified from the fold increase of the translocation time Δ R plotted below the carpets. Negative Δ R values correspond to a decrease of the translocation time. An example for a diffusion barrier that is most pronounced for the 0.6 μm separation distance is marked with an arrowhead. Norm., normalized. Full size image To map the spatial arrangement of regions with fast and slow protein transport, AC- and XC carpets were plotted for GFP 1 measurements in water, nucleus and cytoplasm ( Fig. 3c ). In the cytoplasm and particularly in the nucleus, protein mobility was reduced at a subset of positions. This mobility pattern indicated the presence of diffusion barriers created by inaccessible regions that hinder molecular transport as observed previously using scanning FCS followed by pair-correlation function analysis [13] , [16] , [26] . At the same time, the correlation carpets revealed large regions with high mobility in both cytosol and nucleus, representing extended accessible subcompartments that are separated by barriers. Furthermore, the heterogeneous amplitude values and diffusion times in the correlation carpets of GFP 1 in the nucleus indicate an increased heterogeneity of chromatin compared to the cytoplasmic environment, which is consistent with previous studies [27] , [28] , [29] . Scale-dependent mobility reveals a random obstacle structure We determined the average scale-dependent mobility of GFP 1 , GFP 3 and GFP 5 along a line positioned in the nucleus or cytoplasm to characterize the cellular environment from these proteins’ points of view ( Fig. 4a ). Average AC and XC curves for exemplary distances are shown in Fig. 4b . In the XC curves, a peak was observed at the most frequent translocation time that shifts to larger diffusion times when increasing the separation distances as shown for 1.6 and 3.0 μm. The time dependence of the MSD or the diffusion coefficient retrieved from all XC curves obtained in at least 10 different cells from the human U2OS cell line were evaluated for each GFP multimer type and cellular compartment ( Fig. 5a and Supplementary Note 6 ). The anomalous diffusion behaviour changed from GFP 1 to GFP 5 , revealing a protein size dependence of the accessible cellular space. In general, the overall mobility in the nucleus and the cytoplasm were very similar, suggesting that chromatin and cytosolic obstacles have comparable effects on the translocations of proteins. The time dependence observed for the average diffusion coefficients displayed a sigmoidal shape in double-logarithmic representation. Thus, the cellular environment can be accurately described by a multi-scaling random obstacle organization rather than a single fractal or a corral structure with fixed size ( Fig. 1d ). Figure 4: Measurements on multiple length scales by msFCCS. ( a ) Line-confocal fluorescence images of representative U2OS cells expressing GFP 1 , GFP 3 and GFP 5 . The line positions for the measurement of AC and spatial XC functions in homogeneous regions of the nucleus and cytoplasm are indicated. ( b ) Representative average AC (0 μm) and XC (1.6 and 3 μm) curves obtained in cytoplasm (red) and nucleus (blue). For large diffusion distances, distinct peaks were visible in the diffusion time distributions that shift to larger translocation times for increasing diffusion distance. Solid lines represent the fitted model functions given by Supplementary Equation (22) . Scale bar, 5 μm. Cyt, cytoplasm; Nuc, nucleus; Norm, normalized. 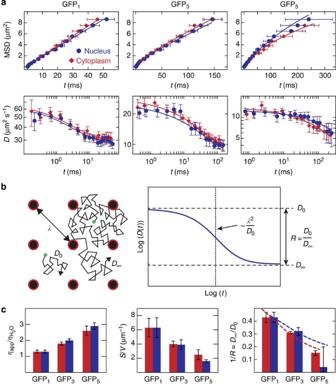Figure 5: Parameters for intracellular topology from time dependence of diffusion coefficients. (a) Average scale-dependent mobility of GFP1(Nuc:n=14 cells, Cyt:n=13 cells), GFP3(Nuc:n=16 cells, Cyt:n=15 cells) and GFP5(Nuc:n=18 cells, Cyt:n=18 cells) in the nucleus and cytoplasm. The time and length scale-dependent protein mobility is represented as the MSD (top row) or as the time-dependent diffusion coefficientD(t) in double-logarithmic representation (bottom row). Data are mean values±s.e.m. The solid lines represent a fit according to the random obstacle model in Equation (1). (b) Time-dependent diffusion coefficients were well described by a model for diffusion in a random porous medium. On small scales, molecules diffuse freely withD0(left). At a characteristic distanceλ, they collide with an immobile obstacle. On large scales, this collision–diffusion process can be described with a reduced diffusion coefficientD∞. The parameters of the model function used for fitting the time-dependent diffusion coefficient in porous media21are illustrated in double-logarithmic representation (right). The initial slope of the curve is related to the surface-to-volume ratioS/V(ref.6). Extrapolation to short time scales yields the microscopic diffusion coefficientD0that would be measured in free solution, and extrapolation to large time scales yields the macroscopic diffusion coefficientD∞for translocations on large length scales. The ratio between both diffusion coefficients is referred to as retardationR. Based on these fit parameters, the correlation lengthλcan be calculated, which represents the length scale above which the medium appears homogeneous if it is sampled by a tracer of a given size. (c) Parameters characterizing the cellular environment derived from the fits of the time-dependent mobility of GFP multimers are the cellular viscosityηapp/ηH2Orelative to water, the surface-to-volume ratioS/Vthat is a measure for the apparent obstacle concentration and the retardationR=D0/D∞. The dependence ofRon the molecule size can be computed for polymeric obstacles to yield estimates for the average fibre diameterdfiberand the obstacle volume fractionΦ0(ref.30). Data are mean values±s.e.m. Dashed lines represent fitted model functions given bySupplementary Equation (34). Full size image Figure 5: Parameters for intracellular topology from time dependence of diffusion coefficients. ( a ) Average scale-dependent mobility of GFP 1 (Nuc: n =14 cells, Cyt: n =13 cells), GFP 3 (Nuc: n =16 cells, Cyt: n =15 cells) and GFP 5 (Nuc: n =18 cells, Cyt: n =18 cells) in the nucleus and cytoplasm. The time and length scale-dependent protein mobility is represented as the MSD (top row) or as the time-dependent diffusion coefficient D ( t ) in double-logarithmic representation (bottom row). Data are mean values±s.e.m. The solid lines represent a fit according to the random obstacle model in Equation (1). ( b ) Time-dependent diffusion coefficients were well described by a model for diffusion in a random porous medium. On small scales, molecules diffuse freely with D 0 (left). At a characteristic distance λ , they collide with an immobile obstacle. On large scales, this collision–diffusion process can be described with a reduced diffusion coefficient D ∞ . The parameters of the model function used for fitting the time-dependent diffusion coefficient in porous media [21] are illustrated in double-logarithmic representation (right). The initial slope of the curve is related to the surface-to-volume ratio S / V (ref. 6 ). Extrapolation to short time scales yields the microscopic diffusion coefficient D 0 that would be measured in free solution, and extrapolation to large time scales yields the macroscopic diffusion coefficient D ∞ for translocations on large length scales. The ratio between both diffusion coefficients is referred to as retardation R . Based on these fit parameters, the correlation length λ can be calculated, which represents the length scale above which the medium appears homogeneous if it is sampled by a tracer of a given size. ( c ) Parameters characterizing the cellular environment derived from the fits of the time-dependent mobility of GFP multimers are the cellular viscosity η app / η H 2 O relative to water, the surface-to-volume ratio S / V that is a measure for the apparent obstacle concentration and the retardation R = D 0 / D ∞ . The dependence of R on the molecule size can be computed for polymeric obstacles to yield estimates for the average fibre diameter d fiber and the obstacle volume fraction Φ 0 (ref. 30 ). Data are mean values±s.e.m. Dashed lines represent fitted model functions given by Supplementary Equation (34) . Full size image msFCCS retrieves parameters for a porous medium topology The scale-dependent mobility of GFP monomer and multimers shown in Fig. 5a were accurately fitted by a simple model for diffusion in porous media consisting of randomly distributed obstacles [21] . It describes the apparent diffusion coefficient by the following equation: This relation contains the following fit parameters ( Fig. 5b ): (i) The microscopic diffusion coefficient D 0 of the particles observed at short time/length scales that describes their mobility in the absence of collisions with obstacles. (ii) The correlation length λ , which is a measure for the typical distance between obstacles. It is inversely proportional to the surface-to-volume ratio S/V . Since potential binding sites are located at the surface of intracellular structures, the parameter S/V is an important experimental readout for the characterization of target search processes as discussed below. The S / V ratio yields the structure’s surface area that is sensed by diffusing proteins per unit volume ( Supplementary Fig. 7 ). It depends on the volume fraction occupied by the obstacles and their spatial arrangement. For example, diffusing proteins sense less surface area in a clustered obstacle network than in a network of homogeneously distributed obstacles with the same obstacle volume fraction. (iii) The reduced macroscopic diffusion coefficient D ∞ measured at large time/length scales at which the MSD grows linearly with time. The ratio of D 0 / D ∞ yields the retardation coefficient R . On the basis of R and the hydrodynamic radius of the tracer particles, the dimensions of fibre-shaped randomly placed obstacles can be derived according to the approach of Phillips [30] ( Supplementary Note 7 ; Supplementary Fig. 8 ). From the microscopic diffusion coefficient D 0 compared with the diffusion coefficient in water, the apparent viscosity η app of the bulk solution in the cell is obtained for each protein species. The diffusion coefficient determined for GFP 1 in buffer equalled D =88±3 μm 2 s −1 in good agreement with previously reported measurements [28] . The corresponding value in the cell was 1.3-fold lower ( Table 2 ). This reduction reflects the subtle increase of the intrinsic viscosity of the cellular environment ( Fig. 5c ) due to the presence of small soluble factors. Thus, the intrinsic cellular viscosity is very similar to that of an aqueous solution. This agrees very well with previous results on the intracellular viscosity obtained from the rotational diffusion coefficient of GFP 1 (refs 31 , 32 ). For GFP 3 and GFP 5 , the corresponding ratios increase to 1.8 and 2.7, indicating that the apparent viscosity for GFP 3 and GFP 5 is increased due to the presence of particles that appear as immobile obstacles to GFP 1 . Table 2 Summary of the results obtained for the porous medium model. Full size table The obstacle surface per volume S/V was higher for smaller molecules like GFP 1 (radius r H ≈2.8 nm) compared with larger molecules like GFP 5 ( r H ≈7.9 nm). Thus, smaller molecules sample the surface of obstacles and barriers with higher resolution to ‘see’ more details and to access smaller pores and channels than larger molecules. Accordingly, molecules might visit different subsets of sites in dependence of their size, leading to partial unmixing of smaller and larger particles. The domain size that appears as a homogeneous environment to a particle diffusing with D 0 is related to the correlation length λ that scales with the inverse of the obstacle surface per volume S / V and equals 0.8±0.2 μm for GFP 1 ( Fig. 5c , Table 2 ). These regions are likely to represent lacunas with residual obstacles that appear mobile from the perspective of the GFP multimer. For translocation distances similar to λ the collision frequency with an apparently immobile obstacle increases considerably, while for distances above λ the average number of collisions per unit distance becomes constant and the time-dependent diffusion coefficient reaches the plateau value D ∞ ( Fig. 5b ). From the dependence of the retardation ratio R = D 0 / D ∞ on multimer size derived previously [30] , we calculated that the obstacles occupy about Φ 0 ~15% of the cellular space if a polymeric fibre-like structure is assumed ( Fig. 5c ; Supplementary Note 7 ). For this case, we determined a mean obstacle diameter d fiber of about 12±4 nm in the nucleus and 8±4 nm in the cytosol. Cytoskeleton and chromatin perturbations affect GFP mobility To dissect the individual mobility contraints imposed by different cytoskeletal filaments, we conducted mobility measurements in cells treated with different drugs that disrupt the cytoskeleton ( Fig. 6 ). We disassembled actin filaments with cytochalasin D (CYTD) [33] , vimentin filaments with withaferin A (WFA) [34] and microtubules with nocodazole (NOC) [35] . Cytoskeletal filaments were efficiently disrupted as apparent on images acquired before and after drug treatment ( Fig. 6 and Supplementary Fig. 9 ). Measurements of the time-dependent mobility of GFP 3 by msFCCS revealed moderate effects of cytoskeletal filament disassembly on GFP 3 transport ( Fig. 6 and Table 2 ). On perturbation of actin microfilaments or vimentin filaments, lower retardation values were obtained that are indicative of a reduced obstacle concentration. Interestingly, no significant changes of GFP 3 mobility were observed on disruption of the microtubule network. This suggests that actin and intermediate filaments are the main fibre-shaped cytoskeletal structures that affect diffusion of GFP 3 in the cytoplasm. However, the moderate effects observed here suggest that other cytosolic components also influence molecular transport significantly. 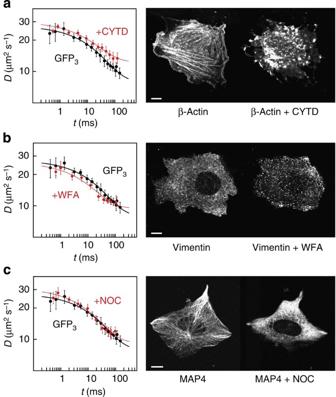Figure 6: Mobility of GFP3in the cytoplasm after disassembly of cytoskeletal filaments. Time-dependent diffusion coefficients measured in U2OS cells after perturbation of the cytoskeleton (red) compared with that in unperturbed cells (black,n=19 cells). (a) Disruption of actin microfilaments by cytochalasin D (n=15 cells). (b) Disruption of vimentin filaments by withaferin A (n=16 cells). (c) Disruption of microtubules by nocodazole (n=14 cells). Data are mean values±s.e.m., fit curves correspond to Equation (1). Perturbations were validated based on the distribution of fluorescently tagged β-actin, vimentin or microtubule-associated protein 4 (MAP4), respectively. Scale bar, 10 μm. Figure 6: Mobility of GFP 3 in the cytoplasm after disassembly of cytoskeletal filaments. Time-dependent diffusion coefficients measured in U2OS cells after perturbation of the cytoskeleton (red) compared with that in unperturbed cells (black, n =19 cells). ( a ) Disruption of actin microfilaments by cytochalasin D ( n =15 cells). ( b ) Disruption of vimentin filaments by withaferin A ( n =16 cells). ( c ) Disruption of microtubules by nocodazole ( n =14 cells). Data are mean values±s.e.m., fit curves correspond to Equation (1). Perturbations were validated based on the distribution of fluorescently tagged β-actin, vimentin or microtubule-associated protein 4 (MAP4), respectively. Scale bar, 10 μm. Full size image To study the impact of chromatin on the mobility of inert particles, cells were treated with the drugs trichostatin A (TSA) [36] , [37] and chloroquine (CQ) [38] . Both substances lead to chromatin decondensation [36] , [37] , [38] , [39] , [40] , [41] by affecting internucleosomal interactions, either via histone hyperacetylation (TSA) or due to DNA intercalation and subsequent changes of DNA twist (CQ). On TSA and CQ treatment, the macrosocpic diffusion coefficient D ∞ of GFP 3 in the nucleus increased and the retardation R decreased ( Fig. 7a,b and Table 2 ). The latter effect reflects a reduced obstacle density and was more pronounced for CQ treatment. 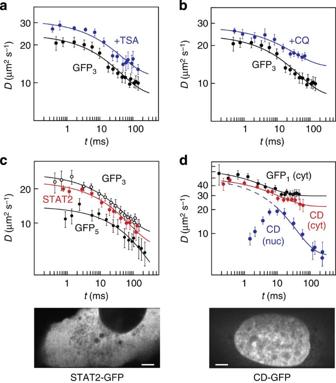Figure 7: Mobility of GFP3in the nucleus after decondensation of chromatin. (a) Time-dependent diffusion coefficient of inert GFP3in the nucleus of U2OS cells after perturbation of the chromatin structure with TSA (blue,n=15 cells) compared with that in unperturbed cells (black,n=16 cells). (b) Same as inabut after perturbation with CQ (blue,n=13 cells). (c) Mobility of STAT2 (red,n=12 cells), GFP3(white,n=15 cells) and GFP5(black,n=18 cells) in the cytoplasm of U2OS cells. The STFM image shows a representative cell expressing GFP-tagged STAT2. (d) Mobility of the chromodomain (CD) of HP1β in the cytoplasm (red,n=11 cells) and nucleus (blue,n=11 cells) compared with that of cytoplasmic GFP1(black,n=13 cells). The STFM image shows a representative cell expressing GFP-tagged CD. Data are mean values±s.e.m., fit curves correspond to Equation (1). Scale bar, 5 μm. Figure 7: Mobility of GFP 3 in the nucleus after decondensation of chromatin. ( a ) Time-dependent diffusion coefficient of inert GFP 3 in the nucleus of U2OS cells after perturbation of the chromatin structure with TSA (blue, n =15 cells) compared with that in unperturbed cells (black, n =16 cells). ( b ) Same as in a but after perturbation with CQ (blue, n =13 cells). ( c ) Mobility of STAT2 (red, n =12 cells), GFP 3 (white, n =15 cells) and GFP 5 (black, n =18 cells) in the cytoplasm of U2OS cells. The STFM image shows a representative cell expressing GFP-tagged STAT2. ( d ) Mobility of the chromodomain (CD) of HP1β in the cytoplasm (red, n =11 cells) and nucleus (blue, n =11 cells) compared with that of cytoplasmic GFP 1 (black, n =13 cells). The STFM image shows a representative cell expressing GFP-tagged CD. Data are mean values±s.e.m., fit curves correspond to Equation (1). Scale bar, 5 μm. Full size image Collisions and binding interactions are dissected by msFCCS To compare the mobility of inert GFP multimers to that of endogeneous proteins, we measured the time-dependent diffusion coefficient for fusion proteins in the nucleus and the cytoplasm. First, we studied the mobility of STAT2–GFP, which is mostly a cytoplasmic protein that accumulates in the nucleus on stimulation to activate a subset of target genes [42] , [43] . Although STAT2–GFP has a molecular weight similar to GFP 5 , its microscopic diffusion coefficient was significantly larger and very similar to that of GFP 3 ( Fig. 7c and Table 2 ). This is in line with the expectation that STAT2–GFP has a more globular structure than the rod-like shaped GFP 5 [27] . Apart from its inherently different shape, STAT2 sensed the cytoplasmic environment just like an inert tracer protein as apparent from its retardation and surface-to-volume ratio ( Table 2 ). The comparison of STAT2–GFP, GFP 3 and GFP 5 demonstrates that the structural parameters obtained from the analysis of GFP multimers reflect the properties of the cellular interior as it is sensed by endogenous proteins. Thus, potential mobility differences arise from additional binding interactions with immobile obstacles in the cell. To further dissect the contribution of obstacle collisions and binding events by msFCCS, we measured the mobility of a well-studied chromatin-interacting protein domain, the chromdomain of HP1β fused to GFP (CD–GFP). It has a molecular weight comparable to inert GFP 1 and binds to histone H3 molecules that carry a trimethylation modification at lysine 9 (ref. 44 ). For CD–GFP, the apparent time-dependent diffusion coefficient was determined in the nucleus and in the cytoplasm. As demonstrated above, both compartments impose similar constraints on the mobility of small molecules ( Fig. 5 ), but the cytoplasm should be devoid of interaction partners of CD–GFP. As expected, the mobility of CD–GFP resembled that of GFP 1 in the cytoplasm ( Fig. 7d ). However, in the nucleus, the mobility of CD–GFP was largely different on both small and large scales due to chromatin binding. The structural parameters determined from the time-dependent diffusion coefficient on larger scales were similar to those for an inert GFP protein but with a significantly reduced macroscopic diffusion coefficient compared with similar-sized GFP 1 ( Table 2 ). Thus, transient chromatin binding caused effective macroscopic diffusion behaviour with a reduced diffusion coefficient [45] . Interestingly, the reduced mobility of the bound CD-GFP pool strongly affected the D (t) profile on small time scales. It resulted in a peak at 10 ms that was neither observed for inert proteins nor for CD–GFP in the cytoplasm ( Fig. 7d ). Thus, the msFCCS analysis conducted here allows for following the transition from the reaction-diffusion controlled regime on small scales to effective diffusion behaviour on large scales. Our approach to extract the scale-dependent mobility of proteins by msFCCS and to link it with intracellular architecture provides structural information on the nanometre scale that is given by the size of the GFP tracer molecules. It addresses a number of long-standing questions on how proteins sense the cellular interior that cannot be resolved by methods that operate on single length scales or in fixed cells: (i) The local viscosity of the fluid embedding the cellular content was found to be only 1.3-fold larger than that of water for GFP 1 , consistent with measurements of its rotational diffusion coefficient [31] , [32] . When evaluated over multiple scales, cytoplasm and nucleus imposed similar mobility constraints for particle sizes covered by GFP 1 , GFP 3 and GFP 5 tracers with a slightly higher heterogeneity being present in the nucleus ( Figs 3 and 5 , Table 2 ). These finding are fully consistent with the single-length/time scale measurements conducted previously [27] , [28] , [29] . (ii) Diffusion barriers in both nucleus and cytosol were observed ( Fig. 3 ). Thus, our msFCCS method extends the available repertoire of methods that study changes of molecular transport in the cell due to local structural alterations [13] , [16] , [26] . We found that particles of the size of a GFP pentamer can become trapped as inferred from the distribution of diffusion times in XC carpets ( Fig. 3a ) and we confirmed this finding by FRAP experiments ( Fig. 3b ) on different time scales. (iii) Differently sized and shaped particles with hydrodynamic radii ranging from r H ≈2.8 nm (GFP 1 ) to r H ≈7.9 nm (GFP 5 ) ‘sense’ distinct structural environments with different surface-to-volume ratios and correlation lengths. While larger particles diffuse more slowly and become apparently excluded from certain regions, smaller particles can explore their local environment more thoroughly. We anticipate that this size-dependent difference can have a large impact on the target search mechanism and associated cellular functions, a prediction to be tested in dedicated experiments that are beyond the scope of the present study. Interestingly, the accessible cellular space in the nucleus is not a simple fractal, an issue that has been the subject of several previous studies [20] , [46] , [47] , [48] . Rather, the intracellular environment resembles a multi-scale porous medium formed by randomly distributed obstacles. The scale-dependent mobility of inert particles is accurately represented by a simple three-parameter model [21] ( Figs 5 , 6 , 7 ). It describes two normal diffusion modes characterized by the microscopic and macroscopic diffusion coefficients D 0 and D ∞ , respectively, which are connected by a crossover region. Within the latter region between the two diffusion regimes, the time-dependent diffusion coefficient can be approximated by a power law, which allows for retrieving an apparent fractal dimension. However, this approximation is only suitable on a particular length and time scale, and this scale is different for GFP 1 , GFP 3 and GFP 5 . Thus, we find no evidence for an invariant fractal dimension inherent in the architecture of the accessible space of the cell that could consistently explain the transport properties of differently sized particles. This agrees very well with recent simulation results of transport processes in porous media and polymer networks [49] , [50] . (iv) Cytoskeletal actin, tubulin and intermediate filaments have only a moderate impact on protein transport in the cytoplasm as inferred from the effect of their depolymerization ( Fig. 6 , Table 2 ). This suggests that other cytoplasmic components like membrane-enclosed organelles represent obstacles that significantly influence cytoplasmic protein mobility. In contrast, drug-induced chromatin decondensation reduced the retardation of GFP 3 mobility considerably ( Fig. 7a,b , Table 2 ), pointing to the chromatin network as the dominant obstacle towards translocations in the nucleus. When describing chromatin as a polymeric fibre-like obstacle structure we calculated that it occupies about 15% of the cellular space with a mean obstacle diameter of about 12±4 nm ( Fig. 5c ; Supplementary Note 7 ). These values correspond to the known dimensions of open nucleosome chains. For these, a diameter of 11 nm and an occupied volume fraction of ~18% in the nucleus was reported [51] , [52] , [53] . Furthermore, we conclude from our experiments that dynamic changes of the chromatin conformation can globally or locally regulate transport and target search processes in the nucleus. The msFCCS experiments conducted here in living cells are in excellent agreement with our previous conclusions on TSA-induced changes of chromatin conformation and accessibility [36] , [37] . (v) Endogenous proteins that do not interact with immobile obstacles, such as STAT2 in the cytoplasm, displayed time-dependent diffusion coefficients very similar to those of inert GFP multimers ( Fig. 7c,d , Table 2 ). Thus, the cellular interior resembles a porous medium that imposes mobility constraints on all proteins in a size- and shape-dependent manner. We measured S / V =3.3±1.3 μm −1 for STAT2–GFP versus S / V =6.3±1.3 μm −1 for monomeric GFP in the cytoplasm. Thus, the accessible obstacle surface area scanned by the smaller GFP molecule was much larger than that of STAT2–GFP. In the presence of binding interactions with the obstacle scaffold, the time dependence of the apparent diffusion coefficient changed globally. This change is apparent from the comparison of the measurements of the chromatin-interacting HP1β chromodomain in the cytoplasm and the nucleus ( Fig. 7d ). Binding interactions of CD–GFP in the nucleus manifested themselves as a peak of the time-dependent diffusion coefficient, which was caused by slow fluctuations detected by msFCCS on short time scales. These signals might be linked to the confined motion of chromatin-bound CD–GFP molecules [45] , temporal changes in the number of occupied binding sites or fluctuations caused by different photophysical properties of free and bound CD–GFP molecules [54] . We conclude that binding interactions alter the apparent diffusion coefficient in a scale-dependent manner, which can be exploited to study binding reactions by msFCCS. The dynamic compartmentalization mechanism unravelled here is dependent on protein size as reflected in different S / V values for different proteins ( Table 2 ). It might have important implications for the kinetics of enzymatic reactions, the target search process of proteins and the formation of intracellular patterns. In particular, the preference of small enzymes to move inside distinct lacunas accelerates the binding of target sites in their local vicinity [1] , [55] , which represents a simple but highly efficient mechanism to guide enzymatic reactions within a compartment that is not partitioned by membranes. In the nucleus, this mechanism might explain the differential enzymatic activity found in various parts of chromatin that serve distinct functions. One example for such a specialized chromatin domain is the perichromatin compartment [56] consisting of lacunas with reduced chromatin density and increased transcriptional activity. These loci are likely to appear as accessible regions with reduced obstacle concentration from the perspective of the GFP multimers ( Fig. 8 ). In contrast, other chromatin subcompartments like lamina-associated domains [57] or pericentric heterochromatin [58] have an increased chromatin density and might act as obstacles. In the different nuclear domains, crucial enzymatic processes like transcription or recombination function very differently although they involve the same enzymes [59] , [60] . Thus, the size-dependent mobility and localization of proteins like polymerases or chromatin modifiers is an important aspect to establish spatial patterns. For example, the local enrichment or depletion of differently sized complexes with distinct enzymatic activity that range from 100 kDa to several MDa in molecular weight could generate specific patterns of chromatin modifications as discussed recently for histone demethylases [61] . Notably, cells can locally regulate the accessibility to different compartments by compaction and relaxation of their nanostructure as shown here in measurements of nuclear access in dependence of the histone acetylation state that we modulated by TSA treatment [37] . This type of transition from an open to a condensed chromatin structure has been observed during the differentiation of embryonic stem cells, which is accompanied by a reduction of global histone acetylation [62] , [63] . Interestingly, the open chromatin in embryonic stem cells was linked to an altered gene expression profile that is characterized by the low level expression of a large number of genes, referred to as ‘promiscuous transcription’, which likely correlates with an increased mobility and accessibility of protein factors. Furthermore, we found that treatment of cells with the DNA-intercalator CQ—a known drug against malaria [64] —decondensed chromatin and significantly enhanced protein transport within the nucleus. Such chromatin rearrangements naturally occur in response to DNA damage through the action of ATP-dependent chromatin remodellers and have been shown to be important for efficient DNA repair [39] , [40] , [41] , [65] . This suggests a functional link between chromatin architecture, protein transport and genomic stability. Likewise, other DNA intercalators like doxorubicin [66] that are used for anticancer chemotherapies are expected to exert similar effects. The same applies to histone deacetylase inhibitors other than TSA that are used in cancer therapy [67] . Thus, the relation between drug-induced chromatin changes and altered protein transport unravelled here might be relevant to the clinical activities of several drugs in addition to their established mode of action. Accordingly, we anticipate that our approach to identify the internal cellular organization that governs the mobility and interactions of protein factors in living cells will provide new insight into the interplay between structure and function during development and its disease-related deregulation. 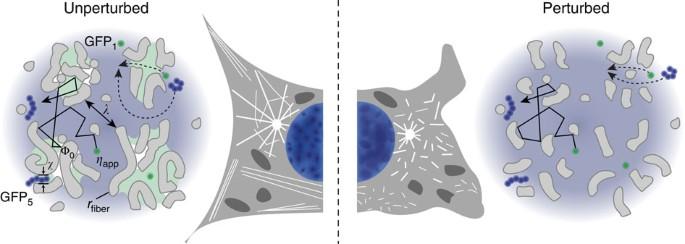Figure 8: The cellular interior appears as a porous medium formed by random obstacles. The correlation lengthλfor the distance between obstacles ‘sensed’ by a given protein is derived from the time dependence of its diffusion coefficient (Fig. 5).The parameterχ~15 nm is the estimated throat size of small pores that confine regions in the nucleus where GFP5(hydrodynamic radiusrH≈7.9 nm) is trapped while GFP3(rH≈5.5 nm) remains mobile. Drug treatment induced structural changes as depicted on the right side of the scheme. Disassembly of cytoplasmic filaments resulted in a moderate increase of GFP3mobility (Fig. 6,Table 2). In contrast, chromatin decondensation increased GFP3mobility considerably (Fig. 7a,b,Table 2). Thus, chromatin is the major obstacle in the nucleus, whereas in the cytoplasm the cytoskeleton represents only one obstacle among others. Figure 8: The cellular interior appears as a porous medium formed by random obstacles. The correlation length λ for the distance between obstacles ‘sensed’ by a given protein is derived from the time dependence of its diffusion coefficient ( Fig. 5 ).The parameter χ ~15 nm is the estimated throat size of small pores that confine regions in the nucleus where GFP 5 (hydrodynamic radius r H ≈7.9 nm) is trapped while GFP 3 ( r H ≈5.5 nm) remains mobile. Drug treatment induced structural changes as depicted on the right side of the scheme. Disassembly of cytoplasmic filaments resulted in a moderate increase of GFP 3 mobility ( Fig. 6 , Table 2 ). In contrast, chromatin decondensation increased GFP 3 mobility considerably ( Fig. 7a,b , Table 2 ). Thus, chromatin is the major obstacle in the nucleus, whereas in the cytoplasm the cytoskeleton represents only one obstacle among others. Full size image Fluorescence microscopy and spectroscopy Imaging and msFCCS measurements were performed with a further developed microscope based on the previously described STFM setup [12] . The STFM continuously illuminates a line-shaped volume in the sample with laser light at 488 nm. To generate this illumination pattern, the Gaussian profile of a laser beam is cropped with a rectangular aperture, and cylindrical lenses are used to generate a laser beam profile that is focused in one direction and parallel in the perpendicular direction. By focusing this beam profile with a high-numerical objective lens into the sample, a line-shaped illumination volume is obtained. Emitted fluorescence signals from multiple detection volumes equally distributed along a line are recorded with a high quantum efficiency EM-CCD camera with 50-μs time resolution (iXon Ultra DU-897, Andor Technology). Fluorescence signals were recorded on a computer. An acousto-optical tunable filter (AOTFnC-400.650, AA Opto-Electronic) was integrated to minimize unintentional bleaching of fluorescence dyes by fine-adjustment of the illuminating laser beam power. For imaging, the illumination laser beam was deflected by a galvanometric mirror (GSI Lumonics) to scan the line in one direction and to acquire two-dimensional regions of interest. Fluorescent samples, cell culture and msFCCS measurements To determine the PSF of the STFM, yellow-green carboxylate-modified FluoSpheres (Molecular Probes) were fixated on poly- L -lysine (Sigma-Aldrich) coated cover slides and subsequently imaged. Alternatively, we used 13-nm-diameter fluorescent QDots with an emission maximum at 525 nm (yellow-green streptavidin conjugated QDots, Invitrogen) as fluctuating point light sources. QDots were immobilized on biotinylated bovine serum albumin coated LabTek chambered coverglasses (Nunc) by incubating a 0.3-nM QDot solution for 1 h. Unbound QDots were removed by rinsing the slides with 1 × PBS buffer and water. The in vitro msFCCS measurements were conducted with a solution of QDots in water or purified GFP in 1 × PBS buffer at concentrations of 20 or 100 nM, respectively. For studies in living cells, plasmids encoding GFP 1 , GFP 3 , GFP 5 [28] , STAT2–GFP or CD–GFP were used. The STAT2–GFP plasmid was constructed by cloning the coding sequence of human STAT2 into a pEGFP-N1 vector backbone (Clontech) via Kpn I and Age I. For the CD–GFP plasmid, the chromodomain of human HP1β (aa 1-69) was cloned into the same vector via Bgl II and Hind III. For the expression of GFPs and GFP-tagged proteins, the respective plasmids were transfected into human U2OS cells (DSMZ, German Collection of Microorganisms and Cell Cultures) with effectene (Qiagen). Cells were cultured in Dulbecco’s Modified Eagle’s Medium supplemented with penicillin–streptomycin and 10% fetal bovine serum at 37 °C and 5% CO 2 . In perturbation experiments, cells were incubated with either 8 μM cytochalasin D for 20 min, 10 μM nocodazole for 30 min, 2 μM withaferin A for 3 h, 400 nM TSA for 18 h or 80 μM CQ for 12 h. Perturbations of the cytoskeleton were validated based on the distribution of overexpressed β-actin-mRFP, mCherry-MAP4 or GFP-vimentin. The FCS/msFCCS measurements were conducted in LabTek chambers with a data acquisition time of 1–3 min per measurement. For living cell experiments 10–20 cells were measured in two or three independent experiments. Only cells that did not change their position significantly during the measurement as judged by pictures taken before and after the experiments were used for the analysis. Measurements were conducted in homogeneous regions of nucleus and cytosol to avoid the influence of large vesicles, nucleoli or membranes that could cause intensity fluctuations. Data processing and spatio-temporal analysis FCS measurements in living cells frequently contain slow signal fluctuations due to external noise and movements of the cell or larger domains within it. In addition, bleaching of fluorescent dyes results in continuously decreasing fluorescence signals ( Fig. 2b ). These low frequency variations of the fluorescence signals were removed after Fast Fourier transformation (FFT) of the raw data ( Supplementary Note 3 ; Supplementary Figs 4, 5 and 6 ). In Fourier space, the envelopes of FFT amplitude spectra were defined as mean values of equally large frequency intervals plus three times the corresponding s.d. These were fitted with an envelope model function for signals without intensity trends given by reference signals acquired for QDots in aqueous solution ( Fig. 2b ). High amplitudes at low FFT frequencies were truncated according to the envelope model function to remove the slow fluctuations, and the truncated FFT spectra were converted back to the time domain. Subsequently, the corrected fluorescence data were analysed by calculating the AC curves of each acquired signal and XC curves of each combination of signals from different detection volumes for a given diffusion distance as described previously [12] . The calculated AC and XC correlation curves were fitted by a model function ( Supplementary Note 4 ). The model function required numerical solution of a double integral, which was accomplished with a multidimensional numerical integration algorithm extension to the GNU Scientific Library (GSL) [68] . Fitting of the non-linear model function to the calculated correlation curves was done with a least-squares minimization algorithm of the GSL. Correlation curves were fitted with self-written software in C++ on a computer cluster. Results of the correlation analysis and least-squares fitting routine were further processed and plotted with MatLab (The MathWorks). How to cite this article: Baum, M. et al. Retrieving the intracellular topology from multi-scale protein mobility mapping in living cells. Nat. Commun. 5:4494 doi: 10.1038/ncomms5494 (2014).